Proliferating versus differentiating stem and cancer cells exhibit distinct midbody-release behaviour The central portion of the midbody, a cytoplasmic bridge between nascent daughter cells at the end of cell division, has generally been thought to be retained by one of the daughter cells, but has, recently, also been shown to be released into the extracellular space. The significance of midbody-retention versus -release is unknown. Here we show, by quantitatively analysing midbody-fate in various cell lines under different growth conditions, that the extent of midbody-release is significantly greater in stem cells than cancer-derived cells. Induction of cell differentiation is accompanied by an increase in midbody-release. Knockdown of the endosomal sorting complex required for transport family members, Alix and tumour-suppressor gene 101, or of their interaction partner, centrosomal protein 55, impairs midbody-release, suggesting mechanistic similarities to abscission. Cells with such impaired midbody-release exhibit enhanced responsiveness to a differentiation stimulus. Taken together, midbody-release emerges as a characteristic feature of cells capable of differentiation. The midbody is a transient structure formed during cytokinesis in animal cells by the ingression of the cleavage furrow [1] , [2] , [3] , [4] . It constitutes a cytoplasmic bridge between the two nascent daughter cells that contains the remnants of the central spindle and the contractile ring [5] , [6] . The central part of the midbody, also called Flemming body, is characterized by a morphologically distinct, electron-dense matrix [7] , [8] , [9] . Abscission, which completes cell division, severs the midbody-bridge, bypassing its central matrix. Consequently, the post-abscission midbody with its characteristic matrix is inherited asymmetrically by one of the daughter cells [10] , [11] , [12] . Until recently, the canonical view was that the post-abscission midbody remains associated with the cell that inherited it [4] , [11] , [12] , [13] . This view has largely been based on the observation of intracellular midbodies in cells in culture, often referred to as 'midbody rings' because of their appearance on analysis of certain midbody markers [11] , [14] , [15] . These internalized post-abscission midbody structures are eventually degraded by autophagy [15] . However, studies on the neuroepithelium in vivo have recently revealed an alternative fate of the midbody after cell division, that is, its release into the extracellular fluid [16] , [17] , [18] . This post-abscission route of the midbody constitutes an irreversible disposal of both, the cytoplasmic and membraneous midbody components from the cell, which is not necessarily true in the case of intracellular degradation. In this context, it is noteworthy that not only components of the cytoskeleton such as central spindle and contractile ring constituents, but also certain membrane components become concentrated at the midbody during cell division. For example, the five-transmembrane-domain protein prominin-1 (CD133) [19] , [20] , [21] , a marker of many somatic stem cells and cancer stem cells [22] , [23] , [24] , is clustered at the central part of the midbody-bridge in neuroepithelial and haematopoietic stem and progenitor cells [17] , [25] , and has been shown to be released from neuroepithelial cells along with midbodies at the onset of neurogenesis in vivo [16] , [17] . Thus, the possibility arises that midbody-release may be associated with changes in cell fate. The existence of midbody-release as an alternative pathway to intracellular degradation of post-abscission midbodies raises three key questions. First, how is midbody-release related to abscission? Second, how do cell types that dispose of midbodies predominantly by release differ from cell types that predominantly degrade midbodies intracellularly? Third, what is the functional significance of midbody-release? Here we have addressed these questions by studying midbody-release versus -retention in various cell types and growth conditions in vitro . We find that midbody-release was greater in stem than cancer cells, and that induction of differentiation enhanced midbody release, and we conclude that midbody release may be a feature of cells that have the ability to commit to differentiation. Midbody-release differs between cell lines To explore how widespread a phenomenon midbody-release is, we subjected the conditioned medium of various cell lines ( Supplementary Table S1 ) to a previously established differential centrifugation protocol [16] , and analysed the resulting four pellets (P1–P4) by immunoblotting for markers of the central region of the midbody, citron rho-interacting kinase (CRIK) [26] , [27] and mitotic kinesin-like protein-1 (MKLP-1) [28] ( Fig. 1 ). In the case of the mouse neural stem cell lines NS-5 and CGR8-NS [29] and the mouse embryonic stem (ES) cell line R1 (ref. 30 ), this revealed a peak of midbody marker-containing particles in the P2 (1,200 g , 20 min) pellet ( Fig. 1a,b ), reminiscent of the midbody-derived P2 particles present in the P2 pellet obtained from mouse embryonic ventricular fluid [16] , [17] . To investigate whether midbody-release can also be observed in primary somatic stem cells, we analysed human haematopoietic stem cells (HSCs) isolated from blood samples of healthy donors. Indeed, also for HSCs, grown either on a mesenchymal stromal cell (MSC) feeder layer or on fibronectin-coated dishes, a peak of midbody marker-containing particles was observed in the P2 pellet, indicative of midbody-release ( Fig. 1c–f ). 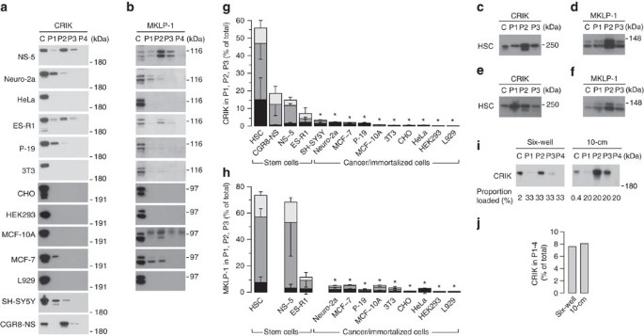Figure 1: Release of membrane particles containing midbody markers from various cell types. Cell lines were grown to subconfluency over a period corresponding to two doubling times, and HSCs were grown for 5 days on MSCs, to condition the respective culture medium. Conditioned media were subjected to differential centrifugation to obtain the P1, P2, P3 and P4 (except for HSCs) pellets. Immunoblots of cell lines (a,b) and of HSCs (c–f) (C, 1/20 of total), and of the corresponding pellets (1/2 of total), for CRIK (a,c,e) and MKLP-1 (b,d,f; same blots as in (a,c,e), respectively, after re-probing). Molecular weight markers are indicated. Quantification of CRIK (g) and MKLP-1 (h) immunoreactivity in the P1 (dark grey), P2 (medium grey) and P3 (light grey) pellets of the indicated cell types, expressed as percentage of total (sum of cells plus P1–4). Data are the mean of three independent experiments, triplicates or quadruplicates (HSCs); bars indicate s.d. Cell types are sorted from left to right in the order of decreasing CRIK immunoreactivity in P1-3. *P⩽0.05, Student'st-test cancer/immortalized cells versus stem cells. CRIK-positive P1-3 particle release between the group of the four stem cells versus ten cancer-derived cells (P-value 0.0005, Student'st-test). (i) CRIK immunoblots of conditioned media of NS-5 cells plated on 6-well plates or 10-cm dishes. The proportion of cells (C) and P1-P4 pellets loaded are indicated. (j) Quantification of CRIK immunoreactivity of the immunoblots shown in (i). The sum of the pellets (P1–4) is expressed as percentage of total (sum of cells plus P1–P4). Figure 1: Release of membrane particles containing midbody markers from various cell types. Cell lines were grown to subconfluency over a period corresponding to two doubling times, and HSCs were grown for 5 days on MSCs, to condition the respective culture medium. Conditioned media were subjected to differential centrifugation to obtain the P1, P2, P3 and P4 (except for HSCs) pellets. Immunoblots of cell lines ( a , b ) and of HSCs ( c – f ) (C, 1/20 of total), and of the corresponding pellets (1/2 of total), for CRIK ( a , c , e ) and MKLP-1 ( b , d , f ; same blots as in ( a , c , e ), respectively, after re-probing). Molecular weight markers are indicated. Quantification of CRIK ( g ) and MKLP-1 ( h ) immunoreactivity in the P1 (dark grey), P2 (medium grey) and P3 (light grey) pellets of the indicated cell types, expressed as percentage of total (sum of cells plus P1–4). Data are the mean of three independent experiments, triplicates or quadruplicates (HSCs); bars indicate s.d. Cell types are sorted from left to right in the order of decreasing CRIK immunoreactivity in P1-3. * P ⩽ 0.05, Student's t -test cancer/immortalized cells versus stem cells. CRIK-positive P1-3 particle release between the group of the four stem cells versus ten cancer-derived cells ( P -value 0.0005, Student's t -test). ( i ) CRIK immunoblots of conditioned media of NS-5 cells plated on 6-well plates or 10-cm dishes. The proportion of cells (C) and P1-P4 pellets loaded are indicated. ( j ) Quantification of CRIK immunoreactivity of the immunoblots shown in ( i ). The sum of the pellets (P1–4) is expressed as percentage of total (sum of cells plus P1–P4). Full size image In contrast, in the case of the tumour-derived Neuro-2a, P-19 and SH-SY5Y cells, the midbody-marker-containing particles in the conditioned medium were largely recovered in the P1 (300 g , 5 min) pellet ( Fig. 1a,b ), indicative of a larger size and/or higher density of these particles (referred to as P1 particles). In the case of the mammary cancer-derived MCF-7 cells and the mammary gland-derived immortalized MCF-10A cells, particles containing MKLP-1 but little CRIK were largely recovered in both the P1 and P2 pellets ( Fig. 1a,b ). Negligible amounts of midbody marker-containing particles were detected in the conditioned medium of various other cancer-derived or immortalized cell lines such as HeLa, NIH-3T3, CHO, HEK293 and L929 cells ( Fig. 1a,b ). We quantified the amount of midbody markers released in particulate form into the culture medium (sum of P1–P4 pellets) after conditioning for a standardized period of time, taking into account the different growth rates of the cell lines studied. This revealed that, relative to the entire culture dish (cells plus conditioned medium), the extent of midbody-marker-containing particles released into the medium was strikingly different between the various cell lines ( Fig. 1g,h ). Interestingly, it was substantially greater for the three stem cell lines NS-5, CGR8-NS and ES-R1 and for HSCs than for the tumour-derived cell lines Neuro-2a, P-19, SH-SY5Y and MCF-7 and the immortalized cell line MCF-10A. Release of CRIK-containing particles for the apparently non-releasing HeLa, 3T3, CHO, HEK293 and L929 cells was <1%. The extent of release of midbody-marker-containing particles was essentially unaffected by the size of the culture dishes used, as observed for NS-5 cells ( Fig. 1i,j ) and HeLa cells analysed for CRIK. As described in Supplementary Note S1 , the midbody-derived extracellular membrane particles in the P1 and P2 pellets were further characterized with regard to their sedimentation properties using velocity sucrose density gradient centrifugation ( Fig. 2 ) and their abundance and morphology by immunofluorescence ( Fig. 3 ). 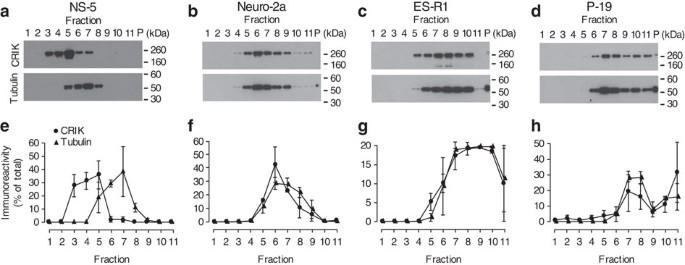Figure 2: Velocity sucrose gradient centrifugation of midbodies released from various cell lines. Conditioned media from NS-5 (a,e), Neuro-2a (b,f), ES-R1 (c,g) and P-19 (d,h) cells were obtained as inFig. 1and subjected to a single centrifugation step to collect the P1 and P2 membrane particles together, which were then subjected to velocity sucrose gradient centrifugation. (a–d) Aliquots of the gradient fractions (1/2 of total, fraction 1=top of gradient) and pellets (P, 1/5 of total) were subjected to immunoblot analysis for CRIK and α-tubulin. The positions of molecular weight markers are indicated. (e–h) Quantification of CRIK (circles) and α-tubulin (triangles) immunoreactivity in the gradient fractions, expressed as percentage of total (sum of gradient fractions). Data are the mean of two independent experiments; bars indicate the variation of the individual values from the mean. Figure 2: Velocity sucrose gradient centrifugation of midbodies released from various cell lines. Conditioned media from NS-5 ( a , e ), Neuro-2a ( b , f ), ES-R1 ( c , g ) and P-19 ( d , h ) cells were obtained as in Fig. 1 and subjected to a single centrifugation step to collect the P1 and P2 membrane particles together, which were then subjected to velocity sucrose gradient centrifugation. ( a – d ) Aliquots of the gradient fractions (1/2 of total, fraction 1=top of gradient) and pellets (P, 1/5 of total) were subjected to immunoblot analysis for CRIK and α-tubulin. The positions of molecular weight markers are indicated. ( e – h ) Quantification of CRIK (circles) and α-tubulin (triangles) immunoreactivity in the gradient fractions, expressed as percentage of total (sum of gradient fractions). Data are the mean of two independent experiments; bars indicate the variation of the individual values from the mean. 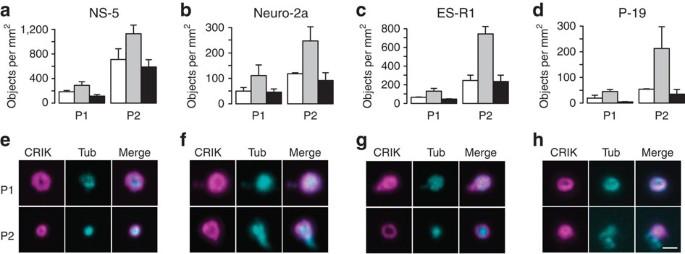Figure 3: Immunofluorescence analysis of midbodies released from various cell lines. Conditioned media from NS-5 (a,e), Neuro-2a (b,f), ES-R1 (c,g) and P-19 (d,h) cells were obtained as inFig. 1and subjected to differential centrifugation to obtain P1 and P2 particles, followed by double immunofluorescence for CRIK and α-tubulin on the cytoplasmic matrix of the particles after sedimentation onto glass coverslips. (a–d) Quantification of objects immunoreactive for CRIK (open columns) and α-tubulin (grey columns) (in either case, values include the CRIK/α-tubulin double-positive objects), and of objects double-immunoreactive for CRIK plus α-tubulin (filled columns), counted in at least six randomly chosen fields. Data are expressed for a coverslip area of one mm2. Data are the mean of two independent experiments; bars indicate the variation of the individual values from the mean. (e–h) Immunofluorescence showing examples of cytoplasmic matrices from P1 and P2 particles double-immunoreactive for CRIK (red) and α-tubulin (blue); note the ring-like appearance of the CRIK immunostaining. Scale bar, 1 μm. Full size image Figure 3: Immunofluorescence analysis of midbodies released from various cell lines. Conditioned media from NS-5 ( a , e ), Neuro-2a ( b , f ), ES-R1 ( c , g ) and P-19 ( d , h ) cells were obtained as in Fig. 1 and subjected to differential centrifugation to obtain P1 and P2 particles, followed by double immunofluorescence for CRIK and α-tubulin on the cytoplasmic matrix of the particles after sedimentation onto glass coverslips. ( a – d ) Quantification of objects immunoreactive for CRIK (open columns) and α-tubulin (grey columns) (in either case, values include the CRIK/α-tubulin double-positive objects), and of objects double-immunoreactive for CRIK plus α-tubulin (filled columns), counted in at least six randomly chosen fields. Data are expressed for a coverslip area of one mm 2 . Data are the mean of two independent experiments; bars indicate the variation of the individual values from the mean. ( e – h ) Immunofluorescence showing examples of cytoplasmic matrices from P1 and P2 particles double-immunoreactive for CRIK (red) and α-tubulin (blue); note the ring-like appearance of the CRIK immunostaining. Scale bar, 1 μm. Full size image Midbody-retention varies between cell lines The number of midbodies formed reflects the rate of cell proliferation. We investigated the extent of midbody-retention in some of the cell lines to explore whether it correlates inversely with midbody-release. Immunofluorescence for CRIK ( Fig. 4a ) and MKLP-1 ( Fig. 4b ) revealed that the proportion of cells with immunoreactive puncta, suggestive of cell-associated midbodies, was greater for HeLa cells, which showed very little midbody-release ( Fig. 1 ), than NS-5 cells, which exhibited a high extent of midbody-release ( Figs 1 and 3 ). Neuro-2a cells displayed an intermediate number of residual midbodies per cell, consistent with the intermediate level of midbody-release ( Figs 1 and 3 ). Quantification of cell-associated CRIK-immunostained midbodies in six of the cell lines analysed for midbody-release in Figure 1 indicated that the average number of residual midbodies per cell ranged from 0.1 to 0.5 ( Fig. 4c ), with the values for NS-5 (0.1) and HeLa (0.4) cells being consistent with an inverse correlation between midbody-release and retention in these cells ( Supplementary Note S2 for the other cell lines). 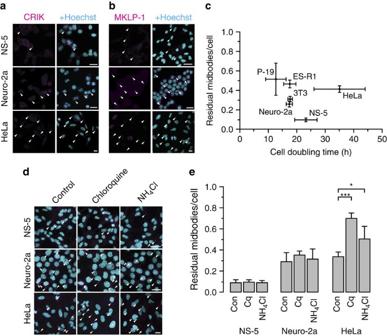Figure 4: Midbody-retention in relation to cell growth rates and in response to inhibition of autophagy. (a,b) Immunofluorescence (red) of NS-5, Neuro-2a and HeLa cells for CRIK (a) and MKLP-1 (b); nuclei were counterstained with Hoechst (blue). Arrowheads indicate residual midbodies in cells; note the greater frequency of residual midbodies in HeLa over Neuro-2a over NS-5 cells. Scale bars, 20 μm. (c) NS-5, Neuro-2a, HeLa, ES-R1, P-19 and 3T3 cells were cultured under conditions allowing exponential growth. The average number of residual midbodies per cell, determined by CRIK immunofluorescence/Hoechst staining as in (a) and counted for at least 100 cells per cell line and experiment, is plotted as a function of cell doubling time. Data are the mean of three independent experiments; bars indicate s.d.P-values for residual midbodies per cell: NS-5 versus all other cells <0.001 except P-19 (<0.05); Neuro-2a versus HeLa and ES-R1 <0.01; 3T3 versus HeLa and ES-R1 <0.05 (Student'st-test). (d,e) NS-5, Neuro-2a and HeLa cells were grown for 3 days in the absence (control, con) and presence of 10 μM chloroquine (Cq) or 1 mM ammonium chloride (NH4Cl). (d) Immunofluorescence (red) for CRIK; nuclei were counterstained with Hoechst (blue). Arrowheads indicate residual midbodies in cells; note the greater frequency of residual midbodies in HeLa, but not NS-5, cells on inhibition of autophagy. Scale bars, 20 μm. (e) Quantification of the average number of residual midbodies per cell, determined by CRIK immunofluorescence/Hoechst staining as in (d) and counted for at least 100 cells per cell line, condition and experiment. Data are the mean of three independent experiments each; bars indicate s.d. *P=0.03; ***P<0.001 (Welch two-samplet-test). Figure 4: Midbody-retention in relation to cell growth rates and in response to inhibition of autophagy. ( a , b ) Immunofluorescence (red) of NS-5, Neuro-2a and HeLa cells for CRIK ( a ) and MKLP-1 ( b ); nuclei were counterstained with Hoechst (blue). Arrowheads indicate residual midbodies in cells; note the greater frequency of residual midbodies in HeLa over Neuro-2a over NS-5 cells. Scale bars, 20 μm. ( c ) NS-5, Neuro-2a, HeLa, ES-R1, P-19 and 3T3 cells were cultured under conditions allowing exponential growth. The average number of residual midbodies per cell, determined by CRIK immunofluorescence/Hoechst staining as in ( a ) and counted for at least 100 cells per cell line and experiment, is plotted as a function of cell doubling time. Data are the mean of three independent experiments; bars indicate s.d. P -values for residual midbodies per cell: NS-5 versus all other cells <0.001 except P-19 (<0.05); Neuro-2a versus HeLa and ES-R1 <0.01; 3T3 versus HeLa and ES-R1 <0.05 (Student's t -test). ( d , e ) NS-5, Neuro-2a and HeLa cells were grown for 3 days in the absence (control, con) and presence of 10 μM chloroquine (Cq) or 1 mM ammonium chloride (NH 4 Cl). ( d ) Immunofluorescence (red) for CRIK; nuclei were counterstained with Hoechst (blue). Arrowheads indicate residual midbodies in cells; note the greater frequency of residual midbodies in HeLa, but not NS-5, cells on inhibition of autophagy. Scale bars, 20 μm. ( e ) Quantification of the average number of residual midbodies per cell, determined by CRIK immunofluorescence/Hoechst staining as in ( d ) and counted for at least 100 cells per cell line, condition and experiment. Data are the mean of three independent experiments each; bars indicate s.d. * P =0.03; *** P <0.001 (Welch two-sample t -test). Full size image The quantification of the average number of residual midbodies per cell ( Fig. 4c ) had been carried out with exponentially growing cells. This allowed us to relate the extent of midbody-retention to cell growth rates. However, no correlation between residual midbody number and cell doubling time was observed for the six cell lines analysed ( Fig. 4c ). Low midbody levels in NS-5 cells are not due to autophagy It has previously been shown that the level of residual midbodies in cells is increased on inhibition of autophagy by drugs neutralizing low-pH compartments, such as chloroquine and ammonium chloride [15] . We, therefore, investigated whether autophagy contributed to the different levels of residual midbodies in NS-5 versus HeLa cells ( Fig. 4a–c ). Cells were treated for 3 days with either 10 μM chloroquine or 1 mM ammonium chloride (higher concentrations were toxic for NS-5 cells) and analysed for cell-associated midbodies by immunofluorescence for CRIK. This revealed that in HeLa cells, inhibition of autophagy resulted in an up to twofold increase in the average level of residual midbodies per cell ( Fig. 4d,e ). In contrast, the low level of residual midbodies in NS-5 cells (as compared with HeLa cells) was unchanged on inhibition of autophagy ( Fig. 4d,e ). We also observed a small (though statistically not significant) increase in residual midbodies in Neuro-2a cells on chloroquine treatment ( Fig. 4d,e ). Ultrastructural aspects of midbody-retention versus -release The data described thus far, together with previous observations [11] , [12] , [14] , [15] , [17] , are consistent with the concept that there are two principal fates of the post-abscission midbody. One is retention by one of the two daughter cells, which predominates in cells such as HeLa, and in which the midbody is typically degraded by autophagy, hence the increase in residual midbodies on inhibition of autophagy. The other is release into the extracellular space, which predominates in cells such as NS-5, and in which the cell-associated stage of the midbody before release does not appear to involve low-pH autophagic organelles. To gain further insight into the membrane processes underlying the distinct fates of the midbody, we analysed the ultrastructure of cell-associated and released midbodies in cells differing in midbody-retention versus -release, using electron microscopy (EM). In HeLa ( Fig. 5a–f ), Neuro-2a ( Fig. 5g–i ) and NS-5 ( Fig. 5j–l ) cells, midbodies before abscission showed the characteristic morphology of their cytoplasm, the clusters of microtubules that represent the remnants of the central spindle, and the electron-dense core in the centre of the midbody that includes the remnants of the contractile ring ( Fig. 5a,g,j ; for serial sections, see Supplementary Fig. S1 ) [4] , [31] . In the subsequent investigation of the ultrastructure of cell-associated versus released midbodies, we shall use the term 'midbody' when both, its characteristic cytoplasmic components and the surrounding plasma membrane, are present. By contrast, we shall use the term 'midbody matrix' for structures containing the characteristic cytoplasmic midbody components but lacking the surrounding plasma membrane. 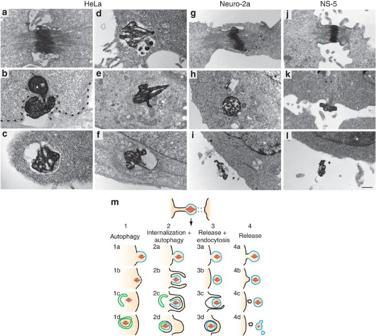Figure 5: EM analysis of midbody-retention and autophagy versus midbody-release. (a–f) HeLa cells, (g–i) Neuro-2a cells, (j–l) NS-5 cells. (a,g,j) Midbodies at telophase. (b) Midbody matrix partially engulfed by one of the daughter cells, before abscission. (c,d) Residual midbodies in intracellular vacuoles of HeLa cells treated with 20 μM chloroquine for three days before fixation; note the longitudinal microtubule bundles. (e,f) Residual midbodies with longitudinal microtubule bundles in intracellular vacuoles of untreated HeLa cells. (h) Residual midbody with cross-sectioned microtubules in an intracellular vacuole of an Neuro-2a cell. (k) Midbody protruding from the surface of an NS-5 cell after abscission. (i,l) Midbodies released from Neuro-2a (i) and NS-5 (l) cells. Nuclei are indicated by asterisks in (e,f,h,i,k,l); asterisk in (b) indicates chromatin, dotted line membrane; scale bar for (a–l), 200 nm. (m) Cartoon illustrating potential fates of the midbody after abscission (top). Pathway 1: the midbody matrix (brown diamond) without midbody plasma membrane (blue) is engulfed by an autophagic vesicle (green). Pathway 2: the midbody (matrix plus plasma membrane) remains attached to one daughter cell and is internalized followed by fusion with an autophagic vesicle. Pathway 3: the midbody (matrix plus plasma membrane) is released from the cell by a second, abscission-like, fission event, followed by endocytosis by the same (3c, d) or another (not illustrated) cell. Pathway 4: the midbody (matrix plus plasma membrane) is released from the cell into the extracellular space by a second, abscission-like, fission event, which may be followed by midbody decomposition (4d). Figure 5: EM analysis of midbody-retention and autophagy versus midbody-release. ( a – f ) HeLa cells, ( g – i ) Neuro-2a cells, ( j – l ) NS-5 cells. ( a , g , j ) Midbodies at telophase. ( b ) Midbody matrix partially engulfed by one of the daughter cells, before abscission. ( c , d ) Residual midbodies in intracellular vacuoles of HeLa cells treated with 20 μM chloroquine for three days before fixation; note the longitudinal microtubule bundles. ( e , f ) Residual midbodies with longitudinal microtubule bundles in intracellular vacuoles of untreated HeLa cells. ( h ) Residual midbody with cross-sectioned microtubules in an intracellular vacuole of an Neuro-2a cell. ( k ) Midbody protruding from the surface of an NS-5 cell after abscission. ( i , l ) Midbodies released from Neuro-2a ( i ) and NS-5 ( l ) cells. Nuclei are indicated by asterisks in ( e , f , h , i , k , l ); asterisk in ( b ) indicates chromatin, dotted line membrane; scale bar for ( a – l ), 200 nm. ( m ) Cartoon illustrating potential fates of the midbody after abscission (top). Pathway 1: the midbody matrix (brown diamond) without midbody plasma membrane (blue) is engulfed by an autophagic vesicle (green). Pathway 2: the midbody (matrix plus plasma membrane) remains attached to one daughter cell and is internalized followed by fusion with an autophagic vesicle. Pathway 3: the midbody (matrix plus plasma membrane) is released from the cell by a second, abscission-like, fission event, followed by endocytosis by the same (3c, d) or another (not illustrated) cell. Pathway 4: the midbody (matrix plus plasma membrane) is released from the cell into the extracellular space by a second, abscission-like, fission event, which may be followed by midbody decomposition (4d). Full size image In HeLa cells, the typical fate of the characteristic cytoplasmic midbody structures was to end up in autophagic vacuoles ( Fig. 5c–f ; for serial sections of Fig. 5f , see Supplementary Fig. S2a ). In most instances, the ultrastructural analysis did not allow us to determine whether this fate involved autophagy of the midbody including its plasma membrane ( Fig. 5m , pathway 2) or just of the midbody matrix ( Fig. 5m , pathway 1). In support of pathway 2, we did observe cases in which internalization of the midbody by one of the daughter cells was initiated before abscission ( Fig. 5b ; for serial sections, see Supplementary Fig. S2b ). In contrast, in NS-5 cells, the morphology of the midbody after abscission was distinct, consistent with its typical fate being the release into the medium ( Fig. 5m , pathway 4). Thus, we frequently observed midbodies that protruded from the surface of one of the daughter cells ( Fig. 5k ) and, on serial sectioning, were found to be no longer connected to the other daughter cell ( Supplementary Fig. S3a ). Serial sections of midbodies protruding from the surface of one daughter cell and no longer connected to the other daughter cell are shown for ES-R1 cells in Supplementary Figs S4 and S5 . Moreover, we frequently observed midbodies in the vicinity of the cell surface ( Fig. 5l ) that on serial sectioning were found to be no longer connected to any cell ( Supplementary Fig. S3b ). The ultrastructural appearance of both, the plasma membrane-protruding and the cell-detached midbodies was reminiscent of the 'aged' midbodies released from neuroepithelial cells into the ventricular fluid [17] . In Neuro-2a cells, the typical morphology of the midbody after abscission indicated both, its ending-up in an autophagic vacuole ( Fig. 5h ; Supplementary Fig. S6 ) and its being released into the medium ( Fig. 5i ; Supplementary Fig. S6 ). In general, microtubule structure appeared better preserved in autophagic vacuole-contained than released midbodies. The ultrastructural analysis did not allow us to determine whether the pathway to autophagic vacuoles occurred without cell detachment of the midbody ( Fig. 5m , pathways 1 and 2) or after midbody-release followed by endocytosis ( Fig. 5m , pathway 3). Live imaging of midbody-retention versus -release We sought to directly visualize midbody-retention versus -release by live imaging. To this end, we performed long-term time-lapse video microscopy on BAC-transgenic NS-5, Neuro-2a and HeLa cells expressing an MKLP-1–GFP fusion protein ( Supplementary Fig. S7a ). MKLP-1 is known to localize to the spindle midzone in anaphase and to concentrate at the midbody in telophase [28] , [32] , and the same was observed for the MKLP-1–GFP fusion protein ( Supplementary Fig. S7b ). Accordingly, in MKLP-1–GFP expressing cells, midbodies could be readily identified as GFP-positive dots appearing in telophase ( Supplementary Fig. S7c ), which allowed monitoring their subsequent fate (retention versus release), notably after abscission ( Fig. 6a–c ). 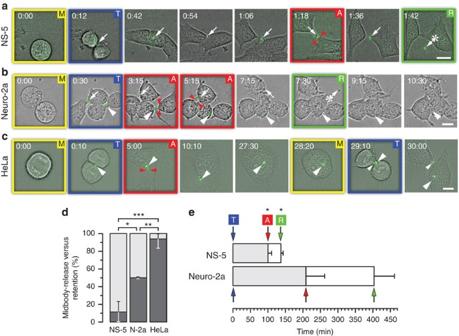Figure 6: Live imaging of the dynamics of midbody-retention versus -release in various cell lines. BAC-transgenic cell lines expressing MKLP-1–GFP were analysed by time-lapse video microscopy for up to 48 h. (a–c) Selected images (combined bright-field and fluorescence) of NS-5 cells (a, 6-min intervals,Supplementary Movie 1), Neuro-2a cells (b, 15-min intervals,Supplementary Movie 3) and HeLa cells (c, 10-min intervals,Supplementary Movie 2); the time points are given as h:min, with the first image shown taken at 6:00 (NS-5), 8:15 (Neuro-2a) and 0:40 (HeLa), respectively, and arbitrarily set to 0:00. Large arrowheads, midbodies destined to be retained; arrows, midbodies destined to be released; arrows with asterisk, released midbodies; small white arrowheads, midbody emerging at second telophase. Yellow frame (M), rounded-up mitotic cell; blue frame (T), cell in telophase with emerging midbody; red frame (A), abscission (double red arrowheads, the last image before the abscission event is shown); green frame (R), midbody-release. Scale bars, 10 μm. (d) Quantification of midbody-release events (light grey) versus midbody-retention events (dark grey), expressed as percentage of total (release plus retention) events in a given experiment. Data are the mean of 3 independent experiments; bars indicate s.d. Number of total events in all experiments together: NS-5, 60; Neuro-2a (N-2a), 50, HeLa, 51. *P=0.02 NS-5 versus Neuro-2a, **P=0.01 Neuro-2a versus HeLa, ***P<0.001 NS-5 versus HeLa (Student'st-test). (e) Determination, for the midbody-release events, of the average time between telophase (blue T and arrows, arbitrarily set to 0 min), abscission (red A and arrows) and midbody-release (green R and arrows) observed in a given experiment. Data are the mean of 3 independent experiments; bars indicate s.d. Asterisks, time from telophase to abscission, and from abscission to midbody-release, between NS-5 and Neuro-2a cells,P-value <0.05. Number of total midbody-release events in all experiments together: NS-5, 52 (the value for abscission was determined from 34 events); Neuro-2a, 32 (Student'st-test). Figure 6: Live imaging of the dynamics of midbody-retention versus -release in various cell lines. BAC-transgenic cell lines expressing MKLP-1–GFP were analysed by time-lapse video microscopy for up to 48 h. ( a – c ) Selected images (combined bright-field and fluorescence) of NS-5 cells ( a , 6-min intervals, Supplementary Movie 1 ), Neuro-2a cells ( b , 15-min intervals, Supplementary Movie 3 ) and HeLa cells ( c , 10-min intervals, Supplementary Movie 2 ); the time points are given as h:min, with the first image shown taken at 6:00 (NS-5), 8:15 (Neuro-2a) and 0:40 (HeLa), respectively, and arbitrarily set to 0:00. Large arrowheads, midbodies destined to be retained; arrows, midbodies destined to be released; arrows with asterisk, released midbodies; small white arrowheads, midbody emerging at second telophase. Yellow frame (M), rounded-up mitotic cell; blue frame (T), cell in telophase with emerging midbody; red frame (A), abscission (double red arrowheads, the last image before the abscission event is shown); green frame (R), midbody-release. Scale bars, 10 μm. ( d ) Quantification of midbody-release events (light grey) versus midbody-retention events (dark grey), expressed as percentage of total (release plus retention) events in a given experiment. Data are the mean of 3 independent experiments; bars indicate s.d. Number of total events in all experiments together: NS-5, 60; Neuro-2a (N-2a), 50, HeLa, 51. * P =0.02 NS-5 versus Neuro-2a, ** P =0.01 Neuro-2a versus HeLa, *** P <0.001 NS-5 versus HeLa (Student's t -test). ( e ) Determination, for the midbody-release events, of the average time between telophase (blue T and arrows, arbitrarily set to 0 min), abscission (red A and arrows) and midbody-release (green R and arrows) observed in a given experiment. Data are the mean of 3 independent experiments; bars indicate s.d. Asterisks, time from telophase to abscission, and from abscission to midbody-release, between NS-5 and Neuro-2a cells, P -value <0.05. Number of total midbody-release events in all experiments together: NS-5, 52 (the value for abscission was determined from 34 events); Neuro-2a, 32 (Student's t -test). Full size image Consistent with the abundant presence of midbodies in the conditioned culture medium ( Figs 1 and 3 ), NS-5 cells released midbodies into the medium in the vast majority (≈90%) of cases ( Fig. 6a,d ; Supplementary Movie 1 ). In contrast, HeLa cells almost always (>90% of cases) showed midbody-retention ( Fig. 6c,d ; Supplementary Movie 2 ), defined as persistence of the cell-associated MKLP-1–GFP dot over one cell cycle or its gradual disappearance within the cell during the cell cycle, which presumably reflected its degradation in autophagic vacuoles ( Fig. 5 ). Midbodies retained by HeLa cells that persisted for longer than one cell cycle were not released during the next cell cycle but rather contributed to the presence of multiple midbodies retained by these cells ( Fig. 6c ; Supplementary Movie 2 ), as observed previously by other investigators [12] , [14] . Interestingly, Neuro-2a cells showed an intermediate behaviour, with midbody-release occurring in half of the cases ( Fig. 6b,d ; Supplementary Movie 3 ). This is consistent with the intermediate values obtained for Neuro-2a cells compared with NS-5 and HeLa cells with regard to the abundance of midbodies in conditioned culture medium ( Fig. 1 ) and the increase in residual midbodies in cells on inhibition of autophagy ( Fig. 4d,e ). The temporal relationship between abscission and midbody-release is unknown. We exploited the present live imaging system to determine this temporal relationship for NS-5 and Neuro-2a cells. In both cell types, midbody-release did not coincide with, but occurred significantly after, abscission ( Fig. 6e ). For NS-5 cells, the average lag period between abscission and midbody-release was more than half an hour, with abscission having occurred ∼ 100 min after appearance of the MKLP-1–GFP midbody dot. For Neuro-2a cells, the time periods from midbody appearance to abscission, and from abscission to release, were even longer ( ∼ 200 min each) ( Fig. 6e ). As to the fate of the released midbodies, we noticed that MKLP-1–GFP containing midbodies released from Neuro-2a cells, after a period of movement in the intercellular space, contacted other Neuro-2a cells ( Supplementary Fig. S8a ). Consistent with this, we observed, by EM, midbodies that had been released into the ventricular fluid to be located in the immediate vicinity of coated pits at the ventricular surface of mouse E10.5 neuroepithelial cells ( Supplementary Fig. S8b ). Immunogold labelling for prominin-1 revealed the budding of small membrane vesicles from such midbodies that apparently were internalized via coated pits ( Supplementary Fig. S8c,d ). Midbody-release increases on stem cell differentiation The present evidence for midbody-release in various cell culture systems provided an opportunity towards obtaining clues as to the significance of midbody-retention versus -release. Specifically, we noticed that the cells showing significant midbody-release all are either stem cells capable of undergoing differentiation (NS-5, CGR8-NS, ES-R1, HSCs) [29] , [33] , [34] or tumour-derived cell lines still responsive to differentiating agents (Neuro-2a, P-19, SH-SY5Y) [35] , [36] , [37] . We, therefore, used NS-5 cells, Neuro-2a cells and HSCs to explore whether switching cells from proliferation to differentiation affects the extent of midbody-release. We first compared midbody-release from NS-5 cells grown under expansion conditions to that from NS-5 cells induced to undergo neuronal differentiation, performing immunoblot analysis for CRIK after isolation of P2 particles from the respective conditioned medium. This showed that from 8 h after induction of differentiation onwards, the amount of CRIK-positive P2 particles released into the medium increased with a concomitant decrease in cell-associated CRIK ( Fig. 7a ). In quantitative terms, differentiating NS-5 cells released almost half of the total CRIK into the medium in association with P2 particles during 20 h ( Fig. 7b ). Concomitant with the increase in midbody-release during differentiation, the proportion of NS-5 cells remaining in the cell cycle, as indicated by BrdU incorporation, decreased ( Fig. 7c ). 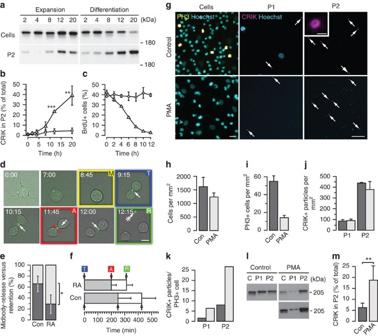Figure 7: Differentiation promotes midbody-release. (a–c) NS-5 cells were cultured in either expansion medium or medium inducing neuronal differentiation, and analysed at the indicated times. (a) CRIK immunoblot of cells (1/10 of total) and P2 pellet of conditioned medium (1/2 of total). (b) Quantification of P2 CRIK immunoblots (circles, expansion; triangles, differentiation) as in (a); total, sum of cells plus P2. Mean of three independent experiments; bars, s.d.P=12 h, ***P<0.001; 20 h, **P=0.004 (Student'st-test) expansion versus differentiation. (c) Percentage of BrdU-labelled cells after 30-min pulse (circles, expansion; triangles, differentiation). Mean of two independent experiments; bars, variation of individual values from mean. (d–f) Time-lapse video microscopy of control (con) and retinoic acid- (RA) treated MKLP-1–GFP transgenic Neuro-2a cells. (d) Selected images (15-min intervals,Supplementary Movie 4) of cell division (RA); time, h:min; 0:00, beginning of time-lapse. Arrows, midbody; asterisk, release. Yellow M, mitotic cell; blue T, telophase; red A, abscission (red arrowheads); green R, midbody-release. Scale bar, 10 μm. (e) Percentage of midbody-release (light grey) versus midbody-retention (dark grey) events. Mean of 3 independent experiments; bars, s.d. Total events: con 50, RA 69. Con versus RA *P<0.05 (Student'st-test). (f) Time between telophase (blue T, arbitrarily set to 0 min), abscission (red A) and midbody-release (green R). Mean of three independent experiments; bars, s.d. Total midbody-release events: con 13, RA 39. (g–m) Analyses of HSCs and P1/P2 pellets of conditioned medium after 24-h culture on MSCs without (control, con; dark grey) or with PMA (light grey). (g) Phosphohistone H3 immunofluorescence (yellow) of cells and CRIK immunofluorescence (red) of P1/P2; Hoechst (blue), nuclei. Scale bars, 20 μm and 1 μm (inset). (h) Cells per mm2(nuclear counts in 0.2–0.6 mm2); mean of four cultures (duplicates from two separate donors); bars, s.d. (i) Mitotic cells per mm2(phosphohistone H3-positive nuclei in 0.6–0.7 mm2); mean of two separate donors; bars, variation of individual values from mean. (j,k) CRIK-immunoreactive particles in P1/P2 (counting 3–5 random fields as in (g)), expressed per mm2(j) or per phosphohistone H3-positive cell (k); mean of two independent experiments; bars in (j), variation of individual values from mean. (l) CRIK immunoblots of cells (C, 1/10 of total) and total P1/P2. Bottom PMA blot, longer exposure to normalize cells to control. (m) Quantification of P2 CRIK immunoblots as in (l); total, sum of cells plus P1-3. Mean of five values (two donors, duplicate and triplicate); bars, s.d. **P<0.01 (Student'st-test). Figure 7: Differentiation promotes midbody-release. ( a – c ) NS-5 cells were cultured in either expansion medium or medium inducing neuronal differentiation, and analysed at the indicated times. ( a ) CRIK immunoblot of cells (1/10 of total) and P2 pellet of conditioned medium (1/2 of total). ( b ) Quantification of P2 CRIK immunoblots (circles, expansion; triangles, differentiation) as in ( a ); total, sum of cells plus P2. Mean of three independent experiments; bars, s.d. P =12 h, *** P <0.001; 20 h, ** P =0.004 (Student's t -test) expansion versus differentiation. ( c ) Percentage of BrdU-labelled cells after 30-min pulse (circles, expansion; triangles, differentiation). Mean of two independent experiments; bars, variation of individual values from mean. ( d – f ) Time-lapse video microscopy of control (con) and retinoic acid- (RA) treated MKLP-1–GFP transgenic Neuro-2a cells. ( d ) Selected images (15-min intervals, Supplementary Movie 4 ) of cell division (RA); time, h:min; 0:00, beginning of time-lapse. Arrows, midbody; asterisk, release. Yellow M, mitotic cell; blue T, telophase; red A, abscission (red arrowheads); green R, midbody-release. Scale bar, 10 μm. ( e ) Percentage of midbody-release (light grey) versus midbody-retention (dark grey) events. Mean of 3 independent experiments; bars, s.d. Total events: con 50, RA 69. Con versus RA * P <0.05 (Student's t -test). ( f ) Time between telophase (blue T, arbitrarily set to 0 min), abscission (red A) and midbody-release (green R). Mean of three independent experiments; bars, s.d. Total midbody-release events: con 13, RA 39. ( g – m ) Analyses of HSCs and P1/P2 pellets of conditioned medium after 24-h culture on MSCs without (control, con; dark grey) or with PMA (light grey). ( g ) Phosphohistone H3 immunofluorescence (yellow) of cells and CRIK immunofluorescence (red) of P1/P2; Hoechst (blue), nuclei. Scale bars, 20 μm and 1 μm (inset). ( h ) Cells per mm 2 (nuclear counts in 0.2–0.6 mm 2 ); mean of four cultures (duplicates from two separate donors); bars, s.d. ( i ) Mitotic cells per mm 2 (phosphohistone H3-positive nuclei in 0.6–0.7 mm 2 ); mean of two separate donors; bars, variation of individual values from mean. ( j , k ) CRIK-immunoreactive particles in P1/P2 (counting 3–5 random fields as in ( g )), expressed per mm 2 ( j ) or per phosphohistone H3-positive cell ( k ); mean of two independent experiments; bars in ( j ), variation of individual values from mean. ( l ) CRIK immunoblots of cells (C, 1/10 of total) and total P1/P2. Bottom PMA blot, longer exposure to normalize cells to control. ( m ) Quantification of P2 CRIK immunoblots as in ( l ); total, sum of cells plus P1-3. Mean of five values (two donors, duplicate and triplicate); bars, s.d. ** P <0.01 (Student's t -test). Full size image We then used the MKLP-1–GFP-expressing Neuro-2a cells to compare midbody-retention versus -release by time-lapse video microscopy of control cells and cells induced to undergo neuronal differentiation by serum reduction and addition of retinoic acid ( Fig. 7d ; Supplementary Movie 4 ) [36] . Neuronal differentiation of Neuro-2a cells resulted in a twofold increase in midbody-release at the expense of midbody-retention ( Fig. 7e ). In addition, differentiation appeared to reduce the time period between formation of the MKLP-1–GFP midbody dot and abscission, and between abscission and midbody-release ( Fig. 7f ). As a third system to investigate whether switching cells from proliferation to differentiation affects the extent of midbody-release, we compared HSCs grown under control, that is proliferating, conditions to HSCs treated for 24 h with phorbol-12-myristate-13-acetate (PMA), which is known to induce their differentiation [34] ( Fig. 7g–m ). Phorbol ester treatment resulted in a small decrease in cell numbers, as indicated by quantification of nuclei ( Fig. 7g,h ), but caused a massive decrease of cycling HSCs, as indicated by quantification of phosphohistone H3-positive cells ( Fig. 7g,i ). Accordingly, the number of midbodies released into the medium, as indicated by the quantification of CRIK-positive particles in the P1 and P2 pellets, was similar for phorbol-ester-treated HSCs compared with proliferating HSCs when expressed per dish ( Fig. 7j ), but dramatically increased when expressed per mitotic HSC observed at the end of culture ( Fig. 7k ). Consistent with this, the absolute amount of P2-associated CRIK immunoreactivity was similar for phorbol-ester-treated HSCs compared with proliferating HSCs ( Fig. 7l ). Note that most of the CRIK immunoreactivity in the P1 pellet of control HSCs ( Fig. 7l ) reflected non-attached cells rather than P1 particles ( Fig. 7g ). In contrast, the amount of P2-associated CRIK immunoreactivity relative to cellular CRIK immunoreactivity was increased threefold on phorbol ester treatment ( Fig. 7l,m ). In quantitative terms, ∼ 30 midbodies per mitotic HSC observed at the end of culture were released from phorbol-ester-treated HSCs during the 24 h period ( Fig. 7k ). Considering that, first, the cell cycle of HSCs under the present conditions is ∼ 24 h (ref. 34 ) (J.K. and D.C., unpublished data), that is, the HSCs subjected to phorbol ester treatment underwent on average one round of cell division during the culture period, and, second, at any time, one of ∼ 30 cycling HSCs was in mitosis ( Fig. 7h,i , con), these data imply that essentially every cell division of phorbol-ester-treated HSCs was accompanied by midbody-release. As the vast majority of cell divisions of phorbol-ester-treated HSCs give rise to post-mitotic cells ( Fig. 7i ), this, in turn, is consistent with the notion that terminal HSC divisions are associated with midbody-release. Collectively, these observations with three distinct cell systems indicate that switching cells from proliferation to differentiation affects the extent of midbody-release. Specifically, divisions of stem cells and differentiation-responsive tumour cells that result in the production of differentiated progeny, notably terminal divisions, are typically followed by midbody-release, whereas midbody-release occurs less frequently after divisions producing daughter cells that remain in the cell cycle. Role of the abscission machinery in midbody-release From a mechanistic point of view, midbody-release, like abscission, involves plasma membrane fission and hence may utilize core components of the abscission machinery. The endosomal sorting complex required for transport family member, the apoptosis-linked gene 2 interacting protein X (Alix), has previously been shown to be involved in two plasma membrane fission processes, the pinching-off of membrane-enveloped virus particles from the plasma membrane, and abscission [38] , [39] . Alix has been shown to interact with the centrosomal protein 55 (Cep55) and the tumour-suppressor gene 101 (Tsg101) in the latter process [40] . Given that these three proteins are essential components of the abscission machinery, we performed knockdown in NS-5 cells ( Fig. 8a,b ) and MKLP-1–GFP-expressing Neuro-2a cells ( Fig. 8c–n ) by RNAi using small interfering RNAs (siRNAs), and analysed the effects on midbody-release versus retention by immunoblotting for CRIK ( Fig. 8a,b,d,e ) or by quantifying the number of cell-retained midbodies and cells using automated image analysis ( Fig. 8f–j ), respectively. 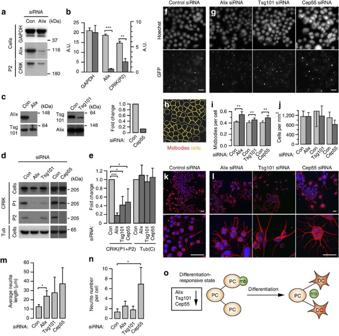Figure 8: RNAi knockdown of abscission machinery affects midbody-release and differentiation. (a,b) NS5-cells were transfected with control (con, light grey) or Alix (dark grey) siRNAs, grown for 2 days, followed by immunoblotting of cells and P2 pellet of conditioned medium. (a) GAPDH and Alix immunoblots of cells (1/20 of total) and CRIK immunoblots of P2 (1/2 of total). (b) Quantification of immunoblots in (a), expressed as arbitrary units (A.U.). Mean of three transfections; bars, s.d. **P<0.01; ***P<0.001 (Student'st-test). (c–n) MKLP-1–GFP transgenic Neuro-2a cells on six-well (c–e), 384-well (f–j) or 24-well (k–n) plates were transfected with control (con, light grey) or Alix, Tsg101 or Cep55 (dark grey) siRNAs, grown for 3 days, and analysed directly (c–j) or after 2 days of differentiation using retinoic acid (k–n). (c) Alix and Tsg101 immunoblots of control and Alix or Tsg101 knockdown cells, and quantitative PCR for Cep55 of control and Cep55 knockdown cells (control set to 1). (d) CRIK and α-tubulin (Tub) immunoblots of control and knockdown cells (C, 1/20 of total) and P1/P2 pellets of 3-day-conditioned medium (1/2 of total). (e) Quantification of immunoblots as in (d), of CRIK in P1+P2 and α-tubulin (Tub) in cells (C), each expressed as fold change of control. Mean of three transfections with one siRNA each; bars, s.d. *P<0.05; ***P<0.001 (Student'st-test). (f,g) Nuclei (Hoechst) and cell-retained midbodies (GFP) of control (f) and knockdown (g) cells. Scale bars, 20 μm. (h) Automated image analysis of control images shown in (f); midbody positions (red) and cell outlines (yellow) obtained from GFP and Hoechst images, respectively. (i,j) Residual midbodies per cell (i) and cells per mm2(j) were calculated from 7–9 images per well using automated image analysis. Mean values of three independent experiments with two siRNAs per target; number of wells analysed per experiment: control, 22; target, 2. Bars, s.d. **P<0.01 (Welch two samplet-test). (k,l) β-III-Tubulin immunofluorescence (red) of control (k) and knockdown (l) cells; blue (Hoechst), nuclei; green (GFP), midbodies. Scale bars, 20 μm. (m,n) Average length (m) and number per cell (n) of neurites were determined from 10 to 30 randomly chosen cells per transfection. Mean of four transfections, using two siRNAs per target; bars, s.d. *P<0.05 (Student'st-test). In total, 70–124 cells were analysed for control and target siRNAs each. (o) Hypothetical relationship between midbody-retention versus -release and differentiation. DC, differentiated cell; mb, midbody; PC, proliferating cell. Figure 8: RNAi knockdown of abscission machinery affects midbody-release and differentiation. ( a , b ) NS5-cells were transfected with control (con, light grey) or Alix (dark grey) siRNAs, grown for 2 days, followed by immunoblotting of cells and P2 pellet of conditioned medium. ( a ) GAPDH and Alix immunoblots of cells (1/20 of total) and CRIK immunoblots of P2 (1/2 of total). ( b ) Quantification of immunoblots in ( a ), expressed as arbitrary units (A.U.). Mean of three transfections; bars, s.d. ** P <0.01; *** P <0.001 (Student's t -test). ( c – n ) MKLP-1–GFP transgenic Neuro-2a cells on six-well ( c – e ), 384-well ( f – j ) or 24-well ( k – n ) plates were transfected with control (con, light grey) or Alix, Tsg101 or Cep55 (dark grey) siRNAs, grown for 3 days, and analysed directly ( c – j ) or after 2 days of differentiation using retinoic acid ( k – n ). ( c ) Alix and Tsg101 immunoblots of control and Alix or Tsg101 knockdown cells, and quantitative PCR for Cep55 of control and Cep55 knockdown cells (control set to 1). ( d ) CRIK and α-tubulin (Tub) immunoblots of control and knockdown cells (C, 1/20 of total) and P1/P2 pellets of 3-day-conditioned medium (1/2 of total). ( e ) Quantification of immunoblots as in ( d ), of CRIK in P1+P2 and α-tubulin (Tub) in cells (C), each expressed as fold change of control. Mean of three transfections with one siRNA each; bars, s.d. * P <0.05; *** P <0.001 (Student's t -test). ( f , g ) Nuclei (Hoechst) and cell-retained midbodies (GFP) of control ( f ) and knockdown ( g ) cells. Scale bars, 20 μm. ( h ) Automated image analysis of control images shown in ( f ); midbody positions (red) and cell outlines (yellow) obtained from GFP and Hoechst images, respectively. ( i , j ) Residual midbodies per cell ( i ) and cells per mm 2 ( j ) were calculated from 7–9 images per well using automated image analysis. Mean values of three independent experiments with two siRNAs per target; number of wells analysed per experiment: control, 22; target, 2. Bars, s.d. ** P <0.01 (Welch two sample t -test). ( k , l ) β-III-Tubulin immunofluorescence (red) of control ( k ) and knockdown ( l ) cells; blue (Hoechst), nuclei; green (GFP), midbodies. Scale bars, 20 μm. ( m , n ) Average length ( m ) and number per cell ( n ) of neurites were determined from 10 to 30 randomly chosen cells per transfection. Mean of four transfections, using two siRNAs per target; bars, s.d. * P <0.05 (Student's t -test). In total, 70–124 cells were analysed for control and target siRNAs each. ( o ) Hypothetical relationship between midbody-retention versus -release and differentiation. DC, differentiated cell; mb, midbody; PC, proliferating cell. Full size image On knockdown of Alix, the amount of CRIK-positive P2 particles released from NS-5 cells into the medium decreased significantly in comparison to control ( Fig. 8a,b ). Similarly, knockdown of Alix, Tsg101 or Cep55 in Neuro-2a cells significantly reduced the amount of CRIK in the P1 and P2 pellets ( Fig. 8c–e ). Accordingly, the number of residual midbodies per cell was significantly increased on Alix, Tsg101 or Cep55 knockdown in Neuro-2a cells compared with control cells ( Fig. 8f,g,i ). By contrast, the number of cells ( Fig. 8j ) was not significantly altered on RNAi for Alix compared with control, suggesting that abscission was not impaired under the present conditions of Alix knockdown. However, knockdown of Tsg101 or Cep55 resulted in a slight (though not statistically significant) reduction in cell number, potentially due to abscission defects. Together, the immunoblotting ( Fig. 8a–e ) and immunofluorescence ( Fig. 8f–j ) data imply that core components of the abscission machinery, notably the endosomal sorting complex required for transport-family member Alix, are also essential factors for midbody-release. Midbody-release impacts on cell differentiation The involvement of Alix, Tsg101 and Cep55 in midbody-release allowed us to test whether knockdown of these proteins would affect the responsiveness of cells to differentiating agents. To this end, we performed siRNA-mediated knockdown in MKLP-1–GFP-expressing Neuro-2a cells, followed by retinoic acid-induced differentiation ( Fig. 8k–n ). Under control conditions ( Fig. 8k ), Neuro-2a cells exposed to retinoic acid typically developed a bipolar morphology, with processes ranging in length from 11 to 16 μm and containing immunoreactivity for βIII-tubulin, a neuronal marker ( Fig. 8k,m,n ). When cells were subjected to Alix RNAi, the average length of processes doubled, ranging from18 to 29 μm ( Fig. 8l,m ). A similar effect was observed on Tsg101 or Cep55 knockdown, although the average length of processes was much more variable and thus its increase not statistically significant ( Fig. 8l,m ). In addition, especially in the case of Cep55, the number of processes per cell was increased on knockdown, with the appearance of large multinucleated cells that occasionally developed a massive outgrowth of highly branched processes ( Fig. 8l ). As an increase in the growth and branching of βIII-tubulin–positive processes of Neuro-2a cells is indicative of their neuronal differentiation [41] , we conclude that knockdown of Alix, Tsg101 or Cep55, which results in reduced midbody-release ( Fig. 8c–j ), also results in increased responsiveness of these cells to a differentiation stimulus. The present study constitutes, to the best of our knowledge, the first quantitative analysis of midbody-release from various cell types. This analysis provides insight into four aspects regarding the release process and its biological significance. First, by comparing different cell types under defined culture conditions, we corroborate the existence of two alternative pathways with regard to the fate of the post-abscission midbody, that is, retention by the daughter cell that inherited it, and release into the extracellular space. The use of these two pathways differed dramatically between distinct cell types and was substantially influenced by the specific growth conditions. Remarkably, midbody-release was highest in neural, haematopoietic and embryonic stem cells and much lower in cancer-derived and immortalized cells. Among the cancer-derived and immortalized cells, it is noteworthy that cell lines still responsive to differentiating agents (Neuro-2a, P-19, SH-SY5Y) showed a greater extent of midbody-release than cell lines lacking this property (for example, HeLa, CHO and HEK293). Although further analyses are clearly required, the present observations raise the exciting possibility that the extent of midbody-release may be related to the differentiation potential of stem and cancer cells. Second, and in line with this possibility, there was an increase in midbody-release at the expense of midbody-retention when NS-5, Neuro-2a cells and HSCs were induced to shift from proliferation to differentiation, that is, to switch their mode of division with regard to the fate of the resulting progeny. In fact, quantification of the number of midbodies released from HSCs on differentiation in relation to the number of cell divisions was consistent with the notion that essentially all divisions giving rise to two post-mitotic daughter cells are accompanied by midbody-release ( Fig. 8o ). The observation that withdrawal from the cell cycle of NS-5 cells subjected to neuronal differentiation is followed by midbody-release supports this notion. In this context, one may speculate about a causal role of midbody-release in cell differentiation. For example, some of the membraneous and cytoplasmic components that cluster at the midbody [4] , [17] , [42] , [43] , [44] may influence the balance between proliferation and differentiation in favour of the former, and, hence, their irreversible removal via midbody-release may contribute to the differentiation of stem and cancer cells. Third, although the timing of midbody-release was found to be different from abscission, the molecular machinery underlying midbody-release was related to abscission. Dissection of the midbody-release process by time-lapse video microscopy of individual cell divisions revealed that midbody-release did not occur concomitant with abscission. Rather, we observed a significant lag period between abscission and midbody-release that varied between the different cell types studied (NS-5, Neuro-2a). This lag period was the shorter the more frequently cells used midbody-release rather than retention (that is, shorter lag in NS-5 compared with Neuro-2a cells, and in retinoic acid-treated compared with control Neuro-2a cells). Importantly, the length of this lag period was not proportional to the duration of the cell cycle, as Neuro-2a cells showed a longer lag period but shorter cell cycle than NS-5 cells. Furthermore, knockdown of Alix, which is known to function in abscission [39] , [45] , or of its interaction partners Tsg101 and Cep55 (ref. 46 ), resulted in a decrease in midbody-release and an increase in midbody-retention. This supports the view that midbody-release, though regulated independently from abscission, is mechanistically related to the latter membrane fission process. In this context, it may be worthwhile to investigate whether CENP-A depleted HeLa cells, which have been reported to exhibit very long and thin midbodies [47] , perhaps exhibit higher midbody-release than the HeLa cells analysed here. Fourth, the identification of Alix, Tsg101 and Cep55 as components of the machinery mediating midbody-release offered an approach to explore a possible link between midbody-release and differentiation. Indeed, knockdown of these proteins in Neuro-2a cells not only increased midbody-retention but also the responsiveness of these cells to a differentiation stimulus, as indicated by the enhanced neurite outgrowth on retinoic acid treatment. These observations are consistent with the hypothesis that, in a proliferating cell capable of responding to a differentiation stimulus, the switch from proliferation to differentiation, notably to terminal divisions of progenitor cells, is accompanied by midbody-release ( Fig. 8o ). Thus, the data presented in the present study provide a basis to further investigate how midbody-retention versus -release and stem/cancer cell proliferation versus differentiation are interrelated. Cell lines Neuro-2a, P-19, SH-SY5Y, HeLa, NIH-3T3, CHO, HEK293 and L929 cells were grown in DMEM supplemented with 10% FCS; MCF-7 were grown in DMEM supplemented with 10% FCS and 1×non-essential amino acids (Sigma); MCF-10A were cultured as described [48] ; ES-R1 (ref. 30 ) in DMEM supplemented with 15% FCS, 2 mM L -glutamine, 1× non-essential amino acids, 100 μM mercaptoethanol and 1,000 U ml −1 LIF (ESGRO, Millipore); NS-5 and CGR8-NS cells in NS cell expansion medium (containing 10 ng ml −1 EGF and 10 ng ml −1 FGF-2) as described [49] . All cell lines were maintained at 37 °C and 5% CO 2 . The MKLP-1 BAC-transgenic cell lines are described in the Supplementary Methods . Culture of cell lines For biochemical experiments, cells were plated on 3-cm dishes at 50,000 (HeLa, P-19), 100,000 (Neuro-2a, 3T3), and 200,000 (NS-5, ES-R1, CHO, HEK293, MCF-7, MCF-10A and L929) cells per dish in 2 ml medium. To determine cell doubling time, cells after 8, 20, 32, 48 and 68 h of growth were removed from the dish and suspended in 1 ml trypsin/EDTA/HBSS, and counted (Kova Glasstic slides). Cell doubling times were calculated from the exponential phases of the growth curves obtained. For some cell lines (CHO, HEK293, MCF-7, MCF-10A and L929), doubling time was estimated by counting cells 24 h after plating and just before centrifugation of the conditioned medium. In the case of SH-SY5Y and CGR8-NS cells, doubling time was estimated from the time that cells split 1:4 or 1:8 and re-plated required to reach the original state of subconfluency. To obtain conditioned medium containing released midbodies, cells were grown for 2 rounds of doubling ( Fig. 1 ), and 1.5 ml of the conditioned medium was collected and subjected to differential centrifugation. Following removal of the remaining medium, cells were lysed on the dish in 200 μl of 2× concentrated SDS sample buffer. For comparing different culture formats, NS-5 cells were plated at 100,000 cells on a six-well plate in 1.5 ml and at 550,000 cells on a 10-cm dish in 10 ml medium. After 48 h, conditioned medium was subjected to differential centrifugation. Cells on six-well plates were lysed in 100 μl, and cells on 10-cm dishes in 550 μl, of 2× SDS sample buffer. For live imaging, cells were plated on gelatin-coated four-well or Lab-Tek eight-well chambered coverglass, at a lower density than for biochemical experiments to facilitate monitoring of individual cells, that is 10,000 cells per cm 2 (NS-5, Neuro-2a) or 5,000 cells per cm 2 (HeLa) in 1 ml and 0.5 ml, respectively, of NS cell expansion medium (NS-5) or DMEM supplemented with 10% FCS (Neuro-2a, HeLa). After 12–24 h, cells were subjected to time-lapse video microscopy. Primary cell culture HSCs and MSCs were collected from healthy donors after informed consent and approval by the local ethics committee. Isolation of MSCs was performed as described [50] . CD34+ MACS-immunoisolated HSCs (300,000 cells) from leukapheresis products [50] were cultured either on fibronectin-coated six-well plates or on MSCs on fibronectin-coated six-well plates, in 3 ml of HSC medium (serum-free medium containing early acting cytokines (50 ng ml −1 stem cell factor, 50 ng ml −1 fetal liver tyrosine kinase-3 ligand, 15 ng ml −1 interleukin-3)) at 37 °C in a humidified 5% CO 2 atmosphere [34] , [50] . To obtain conditioned medium, cells were grown for 5 days, and 1.5 ml of the conditioned medium was subjected to differential centrifugation. Cells were lysed on the dish in 200 μl of 2× concentrated SDS sample buffer. Inhibition of autophagy Cells were plated on coverslips in 3-cm dishes at 50,000 (HeLa) or 200,000 (Neuro-2a, NS-5) cells per dish in 2 ml medium containing 10 μM chloroquine (Sigma) or 1 mM NH 4 Cl, as indicated. After 3 days of growth, cells were fixed and subjected to immunofluorescence. Differentiation of cell lines NS-5 cells were plated on polyornithine-/laminin-coated four-well dishes at 50,000 cells per well in 1 ml NS cell expansion medium. After 15–20 h, the medium was changed to 1 ml of either NS cell expansion medium or medium inducing neuronal differentiation (NS cell expansion medium containing in addition B-27 supplement (Invitrogen) but only 5 ng ml −1 FGF and lacking EGF) [49] . Conditioned medium was collected 30 min after medium change (0 h time point) or 2, 4, 8, 12 and 20 h after the 0 h time point, followed by differential centrifugation. Cells were lysed on the dish in 100 μl of 2× concentrated SDS sample buffer. In BrdU-labelling experiments, NS-5 cells were plated on coverslips and cultured as above, incubated in the presence of 50 μM BrdU for 30 min before the indicated time point, fixed and subjected to BrdU immunofluorescence. Neuro-2a cells were plated on gelatin-coated Lab-Tek four-well or eight-well chambered coverglass at 10,000 cells per cm 2 in 1 ml and 0.5 ml, respectively, of DMEM supplemented with 10% FCS. After 15–20 h, the medium was either replaced with fresh medium (control) or with DMEM supplemented with 2% FCS and 20 μM retinoic acid (dissolved in dimethylsulphoxide (DMSO), final concentration 0.1%) to induce neuronal differentiation, followed by time-lapse video microscopy. In some experiments, Neuro-2a cells were first subjected to RNAi, as described below, followed by differentiation as above for another 2 days, fixation and TuJ-1 immunofluorescence. Differentiation of HSCs HSCs cultured for 3 days were washed with PBS and re-plated (24-well plates) either on fibronectin-coated coverslips or on MSCs on fibronectin-coated coverslips, at 300,000 cells per well in 1 ml of fresh HSC medium. Differentiation medium contained 160 nM PMA(dissolved in DMSO, final concentration 0.01%), whereas control HSC medium contained 0.01% DMSO only. Control dishes with MSCs only indicated lack of contribution of MSCs to the results obtained. Cells on coverslips were kept in control or differentiation HSC medium for 24 h (ref. 34 ). Conditioned medium was collected, followed by differential centrifugation. Cells were lysed on the dish in 100 μl of 2× concentrated SDS sample buffer. Time-lapse video microscopy Cells on chambered coverglass were imaged with a Zeiss Axiovert 200M inverted fluorescence microscope equipped with a motorized stage and incubator, humidifier and carbon dioxide supply (Visitron Systems) to maintain cell culture conditions. Bright-field and fluorescence images were acquired using a C-Apochromat 40× water immersion objective (NA 1.4) and recorded with a Roper Scientific CoolSNAP ES CCD camera using MetaMorph software. For fluorescence, 8–12 z -planes with 0.8–1.5 μm steps were collected at any given time point. Multiple (10–30) fields were imaged in parallel per experiment, using 5–15 min intervals for up to 48 h. In the case of neuronal differentiation of Neuro-2a cells, time-lapse video microscopy was started about 1 h after addition of the retinoic acid-containing medium. RNAi NS-5 cells (six-well plates) were transfected with 250 nM Alix siRNA (Ambion, 5′-GAGGUAUUAUGAUCAGUUTT-3′) or negative control siRNA (Ambion) using Amaxa technology (Lonza, program FP-100, buffer SG). Medium was changed after 1 day and conditioned for 24 h before centrifugation. RNAi of Neuro-2a cells was performed in either an automated manner using a Tecan Freedom Evo 200 liquid handling station (A.W.E., A.-M.M., M.B., A.L. and W.B.H., unpublished results), or conventionally. For automated RNAi, MKLP-1–GFP transgenic Neuro-2a cells were plated on poly- L -lysine-coated 384-well plates in a final volume of 50 μl at 400 cells per well, with each well containing 0.8 μl Interferin (PolyPlus Transfection) and 10 nM siRNA (Invitrogen, Stealth RNAi). For conventional RNAi, transfections in 24- and 6-well plates were scaled up accordingly (24-wells, 5,000 cells, 3.1 μl Interferin, 0.4 ml final volume per well; 6-wells, 50,000 cells, 11 μl Interferin, 1.75 ml final volume per well). Sequences of siRNA oligos were as follows: Alix, 5′-CGGACCUUAAGGAUCUGGAUCCUAU-3′, 5′-UCCAGACUGUCGACCAGCUGAUAAA-3′, Tsg101, 5′-CCAGGCAGAGCUUAAUGCCUUGAAA-3′, 5′-CCCAGUGCGUUAUCGAGGUAAUAUA-3′, Cep55, 5′-UGUCUUCAAGAAGUCCCAAAGAUUU-3′, 5′-GGAACAGCAGAUGCAGGCAUGUACU-3′, negative control siRNA, 5′-UUCCUCUCCACGCGCAGUACAUUUA-3′. Cells in 384-well plates were fixed after 3 days of RNAi and stained with Hoechst 33342. Automated image acquisition was performed using a BD pathway 855 microscope with ×10 objective. Cells in 24-well plates were subjected to RNAi for 3 days and then received fresh medium containing reduced serum and retinoic acid to induce differentiation. Cells in 6-well plates were subjected to RNAi for 3 days followed by immunoblot analysis of cells and medium. Image analysis and quantification Image processing and analysis was done using ImageJ and the ImageJ distribution Fiji ( http://pacific.mpi-cbg.de/wiki/index.php/Fiji ). Z-stacks of images were projected into one plane (maximum intensity projection). Cell-retained midbodies were counted in maximum intensity projections of cells co-stained for α-tubulin to outline the cell borders. In time-lapse video microscopy, telophase cells were defined by the appearance of GFP-positive midbodies. Severing of midbody-bridges, accompanied with a midbody displacement, was taken to indicate abscission events. The midbody of a given cell was followed and scored as released when outside the cell, and as retained when the cell entered the next mitosis with the midbody inside, or when the GFP faded gradually (confirmed by analysing the GFP channel alone). Images of knockdown and control cells were analysed with CellProfiler 2.0 software (The BROAD institute) to determine the number of cells (nuclei) and cell-retained midbodies. Neurite length and number of retinoic acid-differentiated Neuro-2a cells immunostained with TuJ-1 were determined using the Simple Neurite Tracer plug-in of Fiji. Statistical analysis Statistical analysis was performed in 'R' statistical programming environment and Excel (Microsoft). Statistical significance was calculated using Student's t -test or Welch two-sample t -test. How to cite this article: Ettinger, A. W. et al . Proliferating versus differentiating stem and cancer cells exhibit distinct midbody-release behaviour. Nat. Commun. 2:503 doi: 10.1038/ncomms1511 (2011).